Macromolecular structures probed by combining single-shot free-electron laser diffraction with synchrotron coherent X-ray imaging Nanostructures formed from biological macromolecular complexes utilizing the self-assembly properties of smaller building blocks such as DNA and RNA hold promise for many applications, including sensing and drug delivery. New tools are required for their structural characterization. Intense, femtosecond X-ray pulses from X-ray free-electron lasers enable single-shot imaging allowing for instantaneous views of nanostructures at ambient temperatures. When combined judiciously with synchrotron X-rays of a complimentary nature, suitable for observing steady-state features, it is possible to perform ab initio structural investigation. Here we demonstrate a successful combination of femtosecond X-ray single-shot diffraction with an X-ray free-electron laser and coherent diffraction imaging with synchrotron X-rays to provide an insight into the nanostructure formation of a biological macromolecular complex: RNA interference microsponges. This newly introduced multimodal analysis with coherent X-rays can be applied to unveil nano-scale structural motifs from functional nanomaterials or biological nanocomplexes, without requiring a priori knowledge. With its extension of crystallographic methodology to non-crystalline material, the coherent diffraction-imaging (CDI) technique lends support to the unveiling of structures in functional nanomaterial and biological cells and organelles [1] , [2] , [3] , [4] , [5] , [6] , [7] . Imaging of single objects has proven to be a powerful aide in the study of nanostructures, both non-invasively and quantitatively [8] , [9] . Unless a very large number of images is collected, CDI, similar to other imaging probes, may lack in the ability to deliver statistical fidelity, which is particularly crucial to support new scientific discovery. X-ray-scattering techniques, on the other hand, provide faithful statistics, but the data interpretation is contingent on a pertinent model [10] . A structural analysis scheme combining the advantages from each technique is essential for an ab initio understanding of macromolecular complexes, without tangible progress yet. Here we introduce a multimodal coherent X-ray analysis scheme combining X-ray free-electron laser (XFEL) single-shot imaging of single particles, XFEL single-shot small-angle scattering, and coherent diffraction tomography, stereo-imaging and wet CDI using coherent X-rays from synchrotrons [11] . Intense, femtosecond X-ray laser pulses from XFELs have realized single-shot imaging [12] , [13] , [14] , [15] , [16] . This facilitates high-resolution imaging without being limited by radiation damage by capturing diffraction patterns before the onset of radiation-induced structural changes: ‘diffraction-before-destruction’ [17] , [18] . The samples are, however, damaged irreversibly after the single-shot exposure. Synchrotrons, unlike XFELs, supply a quasi-continuous flow of X-ray photons at a lower flux, allowing visualization of the same specimen repeatedly within a manageable time frame. While the image resolution is more severely restricted by the radiation damage when using synchrotron X-rays, the radiation dose can be adjusted conveniently by limiting the exposure time [19] , [20] , [21] , [22] , [23] . We have utilized the unique advantages from each coherent X-ray radiation source, by virtue of their complementary characteristics, to establish a multimodal coherent X-ray analysis scheme, being applied to investigate biomolecular complexes, RNA interference (RNAi) microsponges. The RNAi microsponge was introduced as one of effective delivery systems of small interference RNA (siRNA) molecules [24] , [25] , [26] , [27] , [28] . Without distinguishing cargos and carriers, common in other siRNA delivery systems, the microsponges are formed by self-assembled long RNA molecules containing predetermined RNAi sequences, which can be enzymatically cleaved and converted into siRNA molecules in the cytoplasm after cellular uptake [24] . The efficiency of the programmed double-stranded RNA molecules being diced and converted to siRNA was reported to be 21% [24] . The structure is intrinsically linked to the function, and the knowledge on both internal and external architecture is essential for a complete understanding. However, structural investigation thus far has remained largely focused on surface morphology, making it difficult to understand the formation and disassembly of such functional biomolecules. By employing both imaging and scattering, we investigate the RNAi microsponges from nano-scale details to mesoscopic architecture seamlessly and objectively. This multimodal coherent X-ray analysis scheme, combining XFEL and synchrotron X-rays, unveils a high-density core region within the RNAi microsponge to provide insight into the growth kinetics and suggestion for an improved rational design of the self-assembly. CDI using synchrotron X-rays Nano-scale structures of individual RNAi microsponges were investigated via CDI. We performed CDI experiments at an undulator beamline (BL29XU) in SPring-8. RNAi microsponges of a few micrometers in diameter were dispersed onto a Si 3 N 4 membrane. Sample positions were mapped using an optical microscope before synchrotron X-ray-imaging experiments. We recorded speckle patterns of well-isolated single microsponges using 5 keV X-rays (~3.6 × 10 6 photons s −1 μm −2 ) through a series of short-time (tens of seconds) exposures. Short-exposure diffraction patterns were then compared with each other to monitor any radiation-induced structural alteration, to avoid overexposure to the X-ray radiation. A coherent diffraction pattern was obtained from a ~1.5-μm-sized, air-dried RNAi microsponge displaying oscillatory fringes reflecting the sample size and morphology ( Fig. 1a ). By inverting the diffraction pattern, the image of the specimen was successfully acquired at a pixel scale of 33 nm ( Fig. 1b ). The phase was recovered via an iterative numerical phase retrieval algorithm to render the two-dimensional (2D) projected electron density of the sample (Methods). By estimating the total photon flux, we estimated the density quantitatively as shown by the scale bar to the right (Methods). We then compared the obtained structure with a specimen preserved in a native solution state. A similar diffraction-imaging experiment was performed using specimens mounted in a wet-sample enclosure to acquire an image from a fully hydrated specimen ( Fig. 1c,d ; Methods) [11] . The obtained projection density displays resembling sample morphology and the internal density distribution, similar to the dried sample, supporting that sample’s structure at this resolution is preserved in the dehydrated condition ( Fig. 1b,d ). By confirming that air-dried specimens retain the structural integrity, we have carried out X-ray diffraction experiments under dehydrated conditions with the results introduced hereafter. 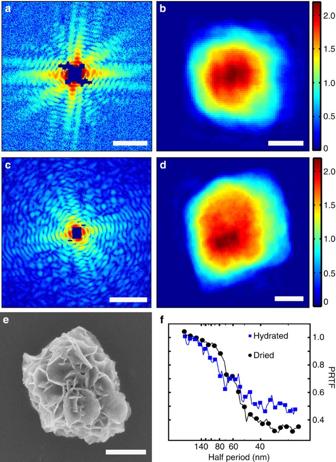Figure 1:Imaging RNAi microsponges with synchrotronX-rays. (a) A speckle pattern is obtained from a dehydrated RNAi microsponge. The dark blue regions represent the portion blocked by the beam stopper and by removing noisy pixel data near the center. (b) The reconstructed image of (a) displays the quantitative density of the RNAi microsponge. (c) A diffraction pattern is recorded from a hydrated RNAi microsponge. (d) Image reconstructed using (c) displays projected density with a high-density core consistent with the dehydrated specimen in (b). The values on the colour bar in (b) and (d) represent 105electrons per nm2. (e) An SEM image taken from a microsponge. No trace for a high-density region can be noticed in the SEM image, visualizing the surface mostly. Scale bars, 5 μm−1(a,c); 500 nm (b,d,e). (f) The phase retrieval transfer function was calculated for the hydrated and dried samples. Figure 1: Imaging RNAi microsponges with synchrotron X-ray s. ( a ) A speckle pattern is obtained from a dehydrated RNAi microsponge. The dark blue regions represent the portion blocked by the beam stopper and by removing noisy pixel data near the center. ( b ) The reconstructed image of ( a ) displays the quantitative density of the RNAi microsponge. ( c ) A diffraction pattern is recorded from a hydrated RNAi microsponge. ( d ) Image reconstructed using ( c ) displays projected density with a high-density core consistent with the dehydrated specimen in ( b ). The values on the colour bar in ( b ) and ( d ) represent 10 5 electrons per nm 2 . ( e ) An SEM image taken from a microsponge. No trace for a high-density region can be noticed in the SEM image, visualizing the surface mostly. Scale bars, 5 μm −1 ( a , c ); 500 nm ( b , d,e ). ( f ) The phase retrieval transfer function was calculated for the hydrated and dried samples. Full size image A scanning electron microscope (SEM) image of a similar RNAi microsponge from the same reaction mixture, representing one of the commonly formed sample morphologies, is shown for comparison ( Fig. 1e ). Distinguished from the flowery surface morphology observed by SEM ( Fig. 1e ), the projection image displays a layered shell-like density distribution, spreading radially, with a high-density region of about 200~300 nm in diameter located near the center ( Fig. 1b,d ; Supplementary Fig. 1 ). The layered density distribution provides evidence that the RNAi microsponge forms a three-dimensional (3D) architecture via progressive packing of molecules; fine-structured layers form a shell-like structure with a dense internal region. The structural consistency observed both in the dried and hydrated microsponges supports that the dense internal region is an intrinsic feature. It, furthermore, ascertains that dehydrated microsponges preserve the native structure of the dense internal core region. The phase retrieval transfer function was calculated to show that the image resolution extends to 70-nm full-period scale ( Fig. 1f ) [14] . We have acquired 2D images of several other single RNAi microsponges confirming that this layered structure is commonly observed ( Supplementary Fig. 2 ). Overall the microsponges are shaped with variations from a spherical shape, some with a more pronounced ellipsoidal feature, but in all cases they are formed compact without having any peculiar extrusion or branches. They share a common radial extension from a higher density inner region, demonstrating the existence of this high-density region irrespective of morphological variation. Stereo-CDI with synchrotron X-rays It is critical to distinguish the density variation in a projection image from differential thickness of the sample. To verify that the high-density core region observed in the projected density is an intrinsic feature, rather than related to sample morphology alone, we have carried out stereo-CDI experiments at SPring-8. The stereo-CDI was realized by taking speckle patterns of the same sample at three different projection angles of +45, 0 and −45° ( Fig. 2a ). Each speckle pattern was then reconstructed independently to exhibit a 2D projection at the corresponding orientation ( Fig. 2b–d ; Supplementary Fig. 3 ). All of the projection images display a high-density region consistently independent of the sample morphology. Using the three projection images, we have deduced the sample architecture ( Fig. 2a ). The 3D shape, inferred from the projections, was introduced as a guide to understand the projected images ( Supplementary Methods ). It displays a localized high-density region independent of sample morphology. The consistency both in the shape and the location of the high-density region clearly exclude the influence from sample thickness, and confirms that a densely compacted core-like structure exists within microsponges ( Fig. 2b–d ). From the three projection images of stereo-CDI, we observed that the core region occupies ~15% of the total projected area and contains ~21% of the total density. 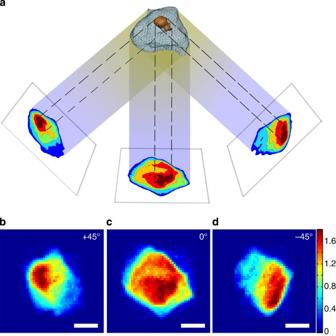Figure 2: Stereo-imaging of an RNAi microsponge. (a) Visualization of projected images with a 3D model. The core region in each projection is highlighted by dotted lines. Density is plotted as a contour map for improved visualization. (b–d) Reconstructed images are shown for the +45°(b), 0°(c) and −45°(d) projections. The electron densities are estimated with the values on the colour bar corresponding to 105electrons per nm2. Scale bars, 500 nm. Figure 2: Stereo-imaging of an RNAi microsponge. ( a ) Visualization of projected images with a 3D model. The core region in each projection is highlighted by dotted lines. Density is plotted as a contour map for improved visualization. ( b – d ) Reconstructed images are shown for the +45 ° ( b ), 0 ° ( c ) and −45 ° ( d ) projections. The electron densities are estimated with the values on the colour bar corresponding to 10 5 electrons per nm 2 . Scale bars, 500 nm. Full size image Quantitative 3D structure using synchrotron X-rays To understand the core-shell-like architecture of RNAi microsponges quantitatively, we have carried out 3D CDI experiments using synchrotron X-rays. A set of speckle patterns was recorded from an isolated RNAi microsponge. The tilt angle was controlled by rotating the sample mounted on a thin solid membrane along an axis perpendicular to the X-ray direction ranging from +69 to −69°. A 3D structure was then reconstructed using 27 projection images ( Fig. 3 ; Methods). 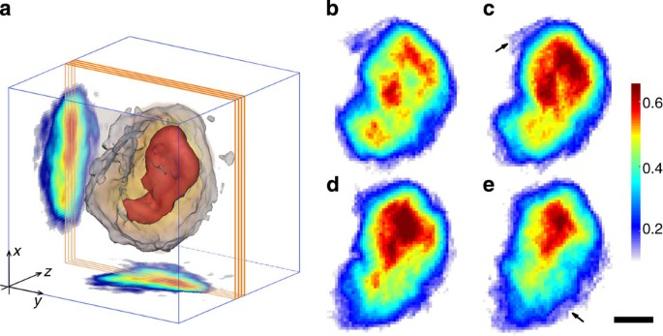Figure 3: 3D architecture of the RNAi microsponge. (a) Complete 3D structure of a microsponge is shown. The sample boundary is displayed transparently (grey) to visualize the internal dense region (red). Projection densities along xz-plane and yz-plane are superposed. (b–e) Sectioned images (xy-planes) clearly distribute the high-density regions inside. The density decreases near the surface and shows extended diffuse layers over 4~5 image pixels, 130~160 nm, inferring the lamella layers (arrows). The position of each sectioned layer is noted in (a) in rectangle (orange); front (b) to back (e) sequence. The direction of incident X-ray is parallel to thezaxis at 0°, and the sample rotation is along thexaxis. Scale bar, 500 nm. The color map on the right shows absolute scale in electrons per Å3. Figure 3: 3D architecture of the RNAi microsponge. ( a ) Complete 3D structure of a microsponge is shown. The sample boundary is displayed transparently (grey) to visualize the internal dense region (red). Projection densities along xz-plane and yz-plane are superposed. ( b – e ) Sectioned images (xy-planes) clearly distribute the high-density regions inside. The density decreases near the surface and shows extended diffuse layers over 4~5 image pixels, 130~160 nm, inferring the lamella layers (arrows). The position of each sectioned layer is noted in ( a ) in rectangle (orange); front ( b ) to back ( e ) sequence. The direction of incident X-ray is parallel to the z axis at 0 ° , and the sample rotation is along the x axis. Scale bar, 500 nm. The color map on the right shows absolute scale in electrons per Å 3 . Full size image The 3D density map displays a dense core region (red) inside the RNAi microsponge via a simplified two-colour representation with the semi-transparently coloured sample surface ( Fig. 3a ; Supplementary Movie 1 ). This core region, representing a region with more rapidly increasing density, shows a higher electron density, 2.3 times of the shell density on average, and occupies ~10% of the total volume, similar to the results deduced from the stereo-imaging ( Figs 2 and 3 ). Individual lamellar-structured layers are not clearly distinguished at this medium image resolution of ~70 nm ( Supplementary Fig. 4 ). However, the 2D images from 65-nm-thin numerical sections show a low-density layer (130~160 nm) towards the sample surface suggesting the presence of porous surface layers consistent with the flowery surface morphology ( Fig. 3b–e ; Supplementary Fig. 5 ). The sliced images are obtained directly from the 3D density by summing two pixel layers, 65-nm-thin slab, along the z-direction ( Fig. 3 ). Quantitative density analysis resulted in an average electron density of 0.54 electrons per Å 3 for the core region and 0.23 electrons per Å 3 for the shell region. The obtained electron density of the core region is close to the nominal value for DNA/RNA of 0.55, implying that it is very tightly packed [29] . The lower density of 0.23 in the shell region, occupying ~90% of the total volume, reflects its highly porous nature to indicate that about 58% of the space in the shell region is empty (Methods). This open area, as the essence of the RNAi microsponges, facilitates their contact with RNase enzymes. Presuming that molecules in the lower density regions have prior access to RNases, the reported efficacy of 21% infers that RNA molecules in the region with the density lower than ~0.19 (blue) would become highly active ( Fig. 3 ). This active region spans ~40% of the total volume in this 3D architecture. It implies that RNase enzyme molecules’ access to about half of the total volume yet remains ineffective. XFEL single-shot imaging using femtosecond X-ray pulses To understand the developmental process of the overall architecture, we have imaged smaller sized, not yet fully formed, RNAi microsponges. We used intense, femtosecond X-ray laser pulses to record discernible speckle patterns from small RNAi microsponges. Synchrotron X-rays could possibly be used. However, in order to compensate for weaker scattering from smaller specimens, much longer exposure time with X-rays is required, which hinders the acquisition of an interpretable diffraction pattern at the desired nano-scale resolution. Thus the single-shot-imaging experiment was performed using the Multiple Application X-ray Imaging Chamber (MAXIC) installed at BL3 of SPring-8 Angstrom Compact free electron LAser (SACLA) [30] , [31] . SACLA was operated with a pulse length of ~10 femtosecond (fs) and a photon energy of 5.5 keV [32] . The pulse energy was 100 μJ at the sample position, with <±7% variation in pulse energy based on the average of 30 pulses. The pulsed X-rays were focused by a pair of K-B mirrors to a 1.5-μm-diameter spot at the focal point, delivering ~1.1 × 10 11 photons in each pulse (~10 GW) [33] . Speckle patterns were obtained through single-shot exposures, now without the influence of radiation-induced distortions. This allows a unique opportunity to compare the intact structure, free of radiation damage, with the images captured by synchrotron X-rays. Samples were mounted on a multi-window Si 3 N 4 membrane [34] . Using a single femtosecond X-ray laser pulse from SACLA, a speckle pattern of an isolated RNAi microsponge of close to 500 × 300 nm in size was recorded ( Fig. 4a ). On retrieving the phase, an image was successfully reconstructed at a significantly improved 17-nm pixel resolution ( Fig. 4b ; Supplementary Fig. 6 ). The quantitative analysis of the electron density bears an uncertainty, compared with the synchrotron experiment, caused mainly by the aforementioned fluctuation in the X-ray pulse energy, but without influencing our interpretation on the core structure here [30] , [35] . As the first single-shot imaging of a biomolecule assembly, this clearly demonstrates the feasibility of obtaining structures from biological complexes including multi-protein complexes and molecular machines through femtosecond single-shot imaging. A high-density region is observed in this small RNAi also, spanning about 5–7 image pixels corresponding to ~80–120 nm, suggesting that the core-like structure is prevalent in these self-assemblies ( Fig. 4b ). An SEM image of a similarly shaped, though much larger, RNAi microsponge is shown ( Fig. 4c ). 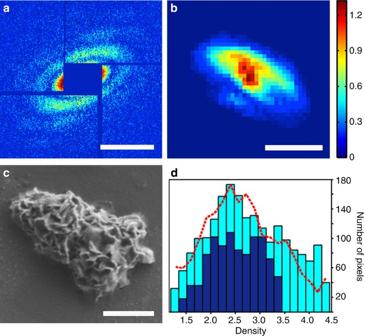Figure 4: Femtosecond single-shot XFEL imaging of an RNA microsponge. (a) A single-shot femtosecond speckle pattern of an RNAi microsponge is obtained at SACLA. (b) Reconstructed image from (a) shows the projected electron density. The colour bar displays the linear density scale in arbitrary unit. (c) An SEM image of a similarly structured, though larger, RNAi microsponge is shown. (d) A histogram of the electron density distribution of the small RNAi (blue) (b) is shown, compared with the density distribution of large RNAi (cyan) (Fig. 1b). The broken red lines represent the average of histograms from large RNAi microsponges imaged at SPring-8 (Supplementary Fig. 2). Scale bar, 10 μm−1, 250 nm and 500 nm (a–c), respectively. Figure 4: Femtosecond single-shot XFEL imaging of an RNA microsponge. ( a ) A single-shot femtosecond speckle pattern of an RNAi microsponge is obtained at SACLA. ( b ) Reconstructed image from ( a ) shows the projected electron density. The colour bar displays the linear density scale in arbitrary unit. ( c ) An SEM image of a similarly structured, though larger, RNAi microsponge is shown. ( d ) A histogram of the electron density distribution of the small RNAi (blue) ( b ) is shown, compared with the density distribution of large RNAi (cyan) ( Fig. 1b ). The broken red lines represent the average of histograms from large RNAi microsponges imaged at SPring-8 ( Supplementary Fig. 2 ). Scale bar, 10 μm −1 , 250 nm and 500 nm ( a – c ), respectively. Full size image To understand its structural resemblance to fully developed RNAi microsponges, the electron density of both small (blue) and large (cyan) RNAi microsponges were compared ( Fig. 4d ). The histogram of the smaller RNAi microsponge displays a similar distribution profile to the larger microsponges. The histograms show an asymmetric distribution of electron density, with a rapid development from the lower density side and slower taper towards higher density. Large RNAi microsponges exhibit a slightly extended density distribution towards higher density. This altogether implies that the high-density core region develops gradually as a result of dynamic compaction of large molecules as the size increases. XFEL single-shot small-angle scattering To statistically support that the observed core-shell-like architecture is a generic feature of RNAi microsponges, coherent small-angle X-ray scattering (cSAXS) was performed. Using femtosecond X-ray laser pulses from SACLA, we have carried out single-shot cSAXS experiments. Instead of an isolated single specimen, now multiple RNAi microsponges were exposed to single femtosecond X-ray pulses. The femtosecond pulses from the XFEL allow SAXS patterns of intact RNAi microsponges to be captured before the onset of radiation damage. Samples were prepared on Si 3 N 4 membrane windows, similar to the single-shot-imaging experiment but at an increased concentration. The experiment was carried out in the MAXIC at BL3 of SACLA with an X-ray energy of 5.5 keV (Methods). A single-shot cSAXS pattern from multiple RNAi microsponges was obtained ( Fig. 5a ). A single-pulse exposure led to a signal that extends across most of the detector area to a spatial resolution of ~6.3 nm with the data extending to 0.16 nm −1 with a good signal-to-noise ratio. We have taken the radial average of the speckle pattern to extract the overall structure of the RNAi microsponges reflected in the small-angle region ( Fig. 5b ). Using information obtained from the observed architecture of the 3D reconstruction, the SAXS pattern was fit to a simplified ellipsoidal core-shell model (red) ( Fig. 5b ). This structure gave a consistent fit to the SAXS data with an error of 0.8%, normalized root mean square (r.m.s.) error, supporting that the core-shell structure is a generic feature in the microsponges ( Fig. 5c ). To further verify the model, we also attempted to fit to a plain ellipsoid without a high-density core shown with the broken blue line ( Fig. 5b ). While this plain ellipsoid may follow the tendency, the fine modulations are simply missed. Many single-shot cSAXS patterns were collected from different single-shot exposures, and exhibit equally good fits to the core-shell structure model ( Supplementary Fig. 7 ). The final fit parameters are summarized in Fig. 5d . The average radii and s.d. of the core and shell sizes in the long and short axes were obtained to be 130 (±50), 100 (±30), 820 (±60) and 650 (±70) nm, respectively. The density of the core estimated from the fit is ~2.4 (±0.3) times of the shell density, consistent with the 3D result. These SAXS results provide strong evidence for the generic existence of the core-shell-like architecture in the RNAi microsponges. 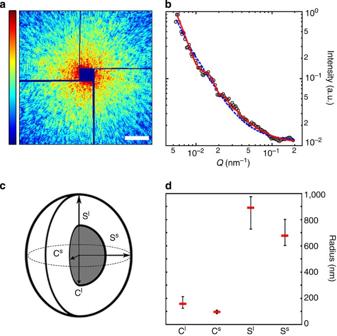Figure 5: XFEL single-shot cSAXS of RNAi microsponges. (a) A femtosecond single-shot speckle pattern is obtained from multiple RNAi microsponges with only the central portion displayed. The colour bar represents the relative intensity, scale bar, 10 μm−1. (b) The radial average of the cSAXS data (circles) is displayed with the fit to the core-shell ellipsoid model (red line) and a plain ellipsoid (blue line). (c) A diagrammatic representation of the core-shell model used for the fit is shown. (d) Results of the fits to a simplified core-shell model are displayed (Cl: core size in a longer axis, CS: core in short, Sl: shell in long and SS: shell in short). The median values are displayed through the center line (red). The error bars (black) show the range of the fit values from different data sets (Supplementary Fig. 7). Figure 5: XFEL single-shot cSAXS of RNAi microsponges. ( a ) A femtosecond single-shot speckle pattern is obtained from multiple RNAi microsponges with only the central portion displayed. The colour bar represents the relative intensity, scale bar, 10 μm −1 . ( b ) The radial average of the cSAXS data (circles) is displayed with the fit to the core-shell ellipsoid model (red line) and a plain ellipsoid (blue line). ( c ) A diagrammatic representation of the core-shell model used for the fit is shown. ( d ) Results of the fits to a simplified core-shell model are displayed (C l : core size in a longer axis, C S : core in short, S l : shell in long and S S : shell in short). The median values are displayed through the center line (red). The error bars (black) show the range of the fit values from different data sets ( Supplementary Fig. 7 ). Full size image The application of the multimodal structure analysis scheme developed here, using coherent X-rays from XFEL and synchrotron sources to RNAi microsponges, reveals that they are oval shaped tessellated structures made of lamella layers extending from a dense core region. The core size is noted to vary in relation to the overall size of the sponge. This, along with the observed density profiles of both large and small microsponges, suggests that this structural motif arises via a dynamic compaction of RNA strands, as the microsponge grows in size. These observations generally support the growth mechanism of the microsponges from densely compacted RNA fibres/sheets, the ‘dense core’ region, with further tessellation of RNA polymers arising from the continued rolling cycle transcription proposed, the ‘tessellation and dynamic packing’, by Lee et al. [24] The crystallinity of the lamella sheet is not directly confirmed in our study without an atomic-scale resolution. Further the 3D architecture of RNAi microsponges helps to better understand the nature and functionality of such self-assembled structures. The 3D density map corresponding to the RNAi microsponges provides profound insight into the self-assembly. The observation that RNA molecules occupying only about 40% of the total volume could be active suggests that the current reported 21% efficacy to generate siRNAs may be improved via better 3D architecture, for example, by growing the microsponges while limiting the core size as much as possible, and reducing the entanglement of the lamellar layers in the porous region. For instance, based on our observations, in particular, of the dense core and decreasing density towards the surface, we may propose the following growth mechanistic to accomplish more cleavable 3D packing of RNA double strands. At first, the growth may be terminated when the nucleation of RNA fibres starts to form, as a way of controlling the core size. Later, these aggregated RNA of nucleation cores can be suspended, as seeds to facilitate tessellation of RNA lamella structures, in fresh solution containing RNA fibres to initiate the microsponge growth without lagging. Under high enough concentration of RNA polymers in a slow growing condition, the radial growth accommodating more effective filling of the space with fibres via branching, nucleation and so on, may be attempted to better utilize the noted empty space, as similarly observed during the formation of bovine insulin amyloid spherulites [36] , [37] , [38] . Here, a controlled growth to produce small-sized microsponges is essential. Smaller RNAi microsponges help to promote easier cellular uptake and to increase the surface-to-volume ratio facilitating active RNA cleavage from the surface. Our study here adds further support with the evidence that the smaller microsponge tends to have a reduced portion of the core region, inferred from the observations of relatively lower ratio in the core-to-shell area in small RNAi microsponges of ~7% compared with larger ones of ~15%, unveiled through the projection densities and similarly from the histogram comparison. The core-shell-like structure of RNAi microsponges, unveiled for the first time from the multimodal analysis of coherent X-rays, may suggest a generic architecture in similar self-assembled biomacromolecules, such as DNA hydrogels, amyloid fibrils and so on [36] , [39] . Long polypeptide chains of biological molecules, similar to polymers, are intrinsically designed to fold to form globular structures to decrease surface energy by increasing molecular bonds [40] . Such self-assembled macromolecular complexes formed from long-chained polymers share similar features of lamellar extensions, radial growth and so on, generally termed as a spherulite [41] . By unveiling the core-shell-like organization within RNAi microsponges, we propose the multimodal coherent X-ray diffraction analysis scheme provides a new route for an in-depth understanding of the spherulite structure as applied to biomolecular complexes. The findings introduced here will encourage further improvement in the rational design of functional biomolecular complexes in general, and deeper understanding of amyloid formation via the approach used here. Nanostructural investigations using coherent X-rays for imaging and scattering analysis have been very active in the last decade, in particular with the increased availability of coherent X-ray sources including X-ray free-electron lasers [6] , [13] , [42] . Intense femtosecond X-ray laser pulses from free-electron lasers have greatly reduced the lower limits on size of single samples that can be investigated. The ‘diffraction-before-destruction’ scheme of the XFEL has introduced a new path to investigate intact structures without radiation-induced sample deformation. However, unveiling a whole 3D structure remains challenging via XFEL single-shot diffraction, especially for non-resembling specimens such as biological cells, biomolecular complexes and so on, where the synchrotron radiation is better suited with quasi-continuous radiation of reduced photon flux. Hence, a multimodal approach judiciously combining such complimentary characteristics is essential, and opens up new capabilities of X-ray structural investigation. In this paper, we demonstrate combined use of tomographic 3D imaging by rotating the same sample, more pertinent with synchrotron X-rays, and single-shot imaging of small specimens at radiation damage unlimited resolution, uniquely available with femtosecond X-ray laser pulses from the XFEL, to gain structural insights from inhomogenous samples [43] , [44] . We propose that the combined applications of synchrotron X-rays and XFELs demonstrated in this work can establish a unique path to seamlessly perform ab initio structure analysis of non-resembling structures within cells, organelles and macromolecular complexes, from micron-scale architectures to nano-scale details. Sample preparation of RNAi microsponges RNAi microsponges were synthesized and purified with a small modification from the method proposed by Lee et al. [24] The circular DNA was prepared by hybridizing a 5′-phosphorylated single-stranded DNA (5′p-ATAGTGAGTCGTATTAACGTACCAACAACTTACGCTGAGTACTTCGATTACTTGAATCGAAGTACTCAGCGTAAGTTTAGAGGCATATCCCT-3′), and a short single-stranded DNA (5′-TAATACGACTCACTATAGGGAT-3′) containing the T7-promoter sequence. A 200-μl reaction mixture containing 1 mM Tris–HCl (pH 8.0) buffer, 20 mM KCl and 0.5 μM of each DNA strand were heated at 95 °C for 2 min, and slowly cooled down to 25 °C over 50 min. The nick in the circular DNA was enzymatically connected by T4 DNA ligase (Promega), and purified by a standard phenol/chloroform extraction and ethanol precipitation. The transcription was performed in a 50-μl reaction mixture containing 40 mM Tris–HCl (pH 8.0), 1 mM spermidine, 5.5 mM MgCl 2 , 10 mM dithiothreitol, 8 mM rNTP’s, 0.1 μM circular DNA template and 5 units μl −1 T7 RNA polymerase (Promega), at 37 °C for 16 h. The resulting solution was centrifuged at 12,000 r.p.m. for 8 min, and the supernatant was discarded. The pellet was then resuspended in 500 μl of RNase-free water, centrifuged and resuspended in the 50 μl of RNase-free water again to remove the excess salt. Data acquisitions at SPring-8 RNAi microsponge samples were first diluted to a suitable concentration, whereby well-isolated microsponges could be located and sonicated for 5 min. Drops (1–3 μl) of the resultant suspension were spread onto a 30-nm-thick Si 3 N 4 membrane (Silson), using a MiTeGen Microloop (MiTeGen) and air-dried. Experiments were performed at BL29XU of SPring-8 with the X-ray energy set at 5 keV. A 10-μm pinhole aperture was used to deliver coherent X-rays to the sample located ~30 cm downstream. Diffraction patterns were recorded on a CCD detector (Roper Inc.) with 1,340 × 1,300 arrays of 20 × 20-μm 2 -sized pixels placed 1.23 m from the samples position. Samples were exposed to X-rays for up to 30 min in short bursts of a few tens of seconds. The speckle pattern used for analysis was obtained by adding all short-exposure patterns. A Si avalanche photodiode was used to monitor the incident X-ray photon flux. Imaging on the fully hydrated RNAi microsponge was carried out by encapsulating the specimens suspended in deionized water using two Si 3 N 4 membranes. This was then further caged in a wet-cell enclosure made of kinematic aluminium plates to hold the two membranes securely, which preserves samples in the solution for over 48 h. Further details of the experimental method can be obtained elsewhere [11] , [45] . The wet-CDI experiments were performed in a helium ambiance using 5 keV X-rays. Data acquisitions at SACLA RNAi microsponges were mounted on Si 3 N 4 membrane similar to SPring-8 experiments for single-shot imaging at SACLA. The membranes were mounted into the MAXIC installed at EH3 of SACLA. Individual XFEL pulses, set at 5.5 keV, were focussed to a size of ~1.5 μm via the K-B mirrors [33] . RNAi microsponges randomly mounted on the membrane were exposed to XFEL pulses by scanning the focused X-ray beams across the membrane window. The resulting diffraction patterns were recorded on a multi-port CCD detector [46] . The multi-port CCD is assembled with eight sensors to give a 2,048 × 2,048 array with 50 × 50 μm 2 size pixels with a 3 × 3-mm 2 central aperture passing the direct beam. Image reconstruction and data analysis Speckle patterns were binned by summing either 3 × 3 or 5 × 5 pixels into one, and then deconvoluted [47] . We used the guided hybrid input-output (GHIO) phase retrieval algorithm to start with 16 random phases for the image reconstruction, with detailed procedures frequently described elsewhere [11] . The single-shot speckle pattern from SACLA was binned by summing 7 × 7 pixels into one. The GHIO was used in a similar manner. The total electron density in the samples (N e ) was estimated using I ( Q=0 )= I 0 r e 2 N e 2 ΔxΔyr −2 , where I 0 is the incident photon flux, r e the classical electron radius, ΔxΔy the area of the central pixel, r the sample to detector distance and I ( Q=0 ) the intensity at the centre pixel, recovered from the measured diffracted intensities [11] . In stereo-imaging, we have modelled a 3D morphology of the sample using the three projection images. The model was deduced using the algebraic reconstruction technique with smoothness ( Supplementary Methods ) [48] . The 3D model from the stereo-imaging is introduced as a guide, and does not suggest a unique solution of the projections. Single-shot cSAXS patterns were radially averaged to generate SAXS patterns. Data were fit to an ellipsoidal core-shell form factor using the SasView program ( http://www.sasview.org/index.html ). The least-square fit was carried out with the radii of the core and shell as parameters. The density of the shell, ~0.25 electrons per Å 3 , was used and the density of the core was allowed to float ( Supplementary Methods ). 3D tomography of a RNAi microsponge The 3D structure was obtained using 27 projections taken at angles fulfilling an equal-slope inclination [49] . First, 2D images were obtained after the phase retrieval of corresponding 2D diffraction patterns using the GHIO algorithm. The data within an array size of 600 × 600 were used for reconstructions. The data were numerically binned by merging 3 × 3 pixel arrays into one pixel enhancing the signal-to-noise ratio by almost an order of magnitude. The numerical deconvolution was then carried out recovering the exactly oversampled diffraction pattern [47] . The final array size of the data used for the GHIO reconstruction became 200 × 200. Details of the GHIO reconstruction procedures can be found elsewhere [11] . All 27 images were obtained following the same procedures. The reconstructions were finished with good fidelity as shown through the phase retrieval transfer function ( Supplementary Fig. 4 ). Using these 27 projection images, we have reconstructed the 3D density map by performing equal-slope tomography (EST) [50] . All 27 projection images were aligned self-consistently to the same rotation center by employing the center-of-mass alignment scheme [51] . The reconstructed images and obtained diffraction patterns were used for the EST reconstructions. The EST allows consistent tomographic reconstruction via iterative refinements of the 3D structure while satisfying the obtained projection images and diffraction patterns simultaneously. Technical details of the EST methods have been published elsewhere [21] , [49] , [52] . The obtained 3D density is visualized by merging the density in 2 × 2 × 2 voxels into one voxel directly without any numerical segmentation ( Fig. 3a ; Supplementary Movie 1 ). The estimated volume fraction of the vacant space (58%) in the shell region was estimated from 1–0.23/0.55, using 0.55 of the nominal RNA density. How to cite this article: Gallagher-Jones, M. et al. Macromolecular structures probed by combining single-shot free-electron laser diffraction with synchrotron coherent X-ray imaging. Nat. Commun. 5:3798 doi: 10.1038/ncomms4798 (2014).